Fate tracing reveals hepatic stellate cells as dominant contributors to liver fibrosis independent of its aetiology Although organ fibrosis causes significant morbidity and mortality in chronic diseases, the lack of detailed knowledge about specific cellular contributors mediating fibrogenesis hampers the design of effective antifibrotic therapies. Different cellular sources, including tissue-resident and bone marrow-derived fibroblasts, pericytes and epithelial cells, have been suggested to give rise to myofibroblasts, but their relative contributions remain controversial, with profound differences between organs and different diseases. Here we employ a novel Cre-transgenic mouse that marks 99% of hepatic stellate cells (HSCs), a liver-specific pericyte population, to demonstrate that HSCs give rise to 82–96% of myofibroblasts in models of toxic, cholestatic and fatty liver disease. Moreover, we exclude that HSCs function as facultative epithelial progenitor cells in the injured liver. On the basis these findings, HSCs should be considered the primary cellular target for antifibrotic therapies across all types of liver disease. Fibrotic diseases account for up to 45% of deaths in developed countries, but we still lack effective antifibrotic therapies [1] . Knowledge about cells contributing to the myofibroblast pool and extracellular matrix (ECM) production in organ fibrosis is important for designing targeted therapies [2] , [3] . Several cell populations, including tissue-resident or bone marrow (BM)-derived fibroblasts, pericytes and epithelial cells, have been suggested as relevant contributors to the myofibroblast pool [2] , [3] , but their contribution varies between organs and different diseases, and remains a matter of debate. Liver fibrosis occurs as a result of chronic liver disease and is associated with severe morbidity and mortality [4] . Hepatic stellate cells (HSCs), a pericyte-like cell population of the liver, and portal fibroblasts are widely considered the most relevant sources of hepatic myofibroblasts, but their precise contribution remains unknown. It is thought that the underlying liver disease determines the cell types that contribute to the myofibroblast pool, with profound differences between toxic and cholestatic liver diseases, and portal fibroblast exerting a key role in the latter [4] , [5] , [6] , [7] . Other cell types such as BM-derived fibrocytes may also contribute to the myofibroblast pool, but to a lesser degree [8] , [9] . However, most evidence about relevant myofibroblast sources and functions derives from cell isolates and in vitro studies [10] , [11] , [12] , whereas in vivo studies quantifying the relative contribution of different cell populations in the fibrotic liver are missing. In this regard, fate-tracing studies have excluded a contribution of hepatocytes and cholangiocytes to the myofibroblast pool [13] , [14] , [15] , but positive identification of cell types contributing to the myofibroblast pool by fate tracing is lacking. As such, previous studies employing collagen-driven Cre or Wt1-Cre have tracked either all collagen-producing myofibroblasts, but not specific cellular sources of myofibroblasts [12] , or mesothelial cells, which give rise to subcapsular fibroblasts within 150 μm of the liver surface but not to intrahepatic myofibroblasts, that is, those that cause organ fibrosis and its deleterious complications [16] . Attempts at fate-tracing HSCs, one of the prime candidates [4] , [11] , [17] , using Cre driven by the human glial fibrillary acidic protein promoter (hGFAPCre) are hampered by the fact that hGFAPCre marks cholangiocytes [18] , [19] ( https://ndp.jax.org/NDPServe.dll?ViewItem?ItemID=1741&XPos=11536496&YPos=5169511&ZPos=0&Lens=1.25&SignIn=Sign%20in%20as%20Guest ), thereby limiting interpretation. Here we employ a novel fate tracing method for HSCs to demonstrate that HSCs are the dominant contributors to collagen-producing myofibroblasts in models of toxic, biliary and fatty liver fibrosis. Moreover, we exclude that HSCs serve as facultative epithelial progenitors in the injured liver. LratCre but not hGFAPCre labels HSCs Using three different Cre reporters, we confirmed that hGFAPCre mice labelled bile ducts and cytokeratin 19-expressing cholangiocytes ( Fig. 1a, e–h ). Of note, hGFAPCre mice did not efficiently mark HSCs or collagen-producing myofibroblasts ( Fig. 1b–g ). Likewise, mice expressing Cre under the murine Gfap promoter did not label HSCs ( Fig. 1i ). To achieve faithful labelling of HSCs, we generated a bacterial artifical chromosome (BAC) transgenic mouse in which Cre expression is driven by lecithin-retinol acyltransferase ( Lrat ; Supplementary Fig. S1B ). Lrat was selected in screens among several candidates because of high expression in HSCs, virtually undetectable expression in hepatocytes, Kupffer cells and cholangiocytes ( Fig. 2a ), and its key role in the formation of retinyl ester-containing lipid droplets, one of the defining features of HSCs [20] . In contrast to a previous study [21] , we also did not detect Lrat protein or messenger RNA expression in endothelial cells ( Fig. 2a ; Supplementary Fig. S1A ). LratCre transgenic mice marked 99% of HSCs as demonstrated by flow cytometry and immunohistochemistry in two different Cre reporter mice, showing nearly complete overlap of HSC markers desmin and Pdgfrβ with LratCre-induced ZsGreen Cre reporter by confocal microscopy, no significant overlap with hepatocyte, macrophage and cholangiocyte markers, and only few spots of overlap with endothelial cell markers, most likely to be due to their very close proximity to HSCs ( Fig. 2b–e and Supplementary Fig. S1C–G ). 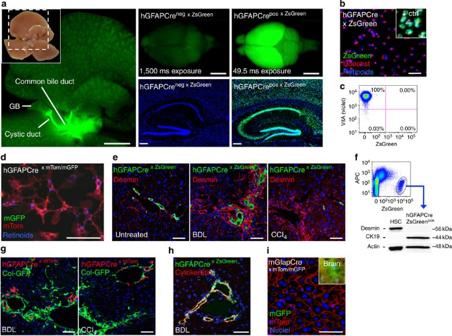Figure 1: GFAPCre marks extra- and intrahepatic bile ducts but not HSCs. (a) Macroscopic images demonstrate hGFAPCre-induced ZsGreen Cre reporter fluorescence in extrahepatic bile ducts, the brain and brain sections (n=1). (b,c) HSCs were isolated from hGFAPCre mice expressing ZsGreen (n=2) and were either plated (b) or analysed by flow cytometry (c). LratCre mice served as positive control (n=3). (d) HSCs were isolated from hGFAPCre mice expressing mTom/mGFP Cre reporter and plated (n=1). (e) Sections from untreated (n=1), bile duct-ligated (n=1) and CCl4-treated livers (n=2) were stained for desmin, showing no co-localization of ZsGreen and HSC marker desmin by confocal microscopy. (f) Representative western blotting (out ofn=3) showing cytokeratin 19 expression but no desmin expression in fluorescence-activated cell sorting-sorted hGFAPCre-labelled ZsGreen-positive cells. (g) hGFAPCre mice undergoing either BDL (n=1) or CCl4treatment (n=1) show no overlap between tdTomato Cre reporter and Col-GFP reporter, thus excluding a contribution of hGFAPCre-labelled cells to ECM-producing myofibroblasts. (h) Cytokeratin staining of bile duct-ligated hGFAPCre mice shows almost complete overlap of cytokeratin, marking the bile duct proliferates, and hGFAPCre-induced ZsGreen expression (n=1). (i) Sections from untreated mice expressing Cre under the murine Gfap promoter and mTom/mGFP Cre reporter show no GFP expression in the liver. The brain served as the positive control (Inlet). Scale bars, 4 mm (a, left panel), 2 mm (a, upper middle and right panel), 200 μm (a, lower middle and right panel) and 50 μm (b,d,e,g–i). Figure 1: GFAPCre marks extra- and intrahepatic bile ducts but not HSCs. ( a ) Macroscopic images demonstrate hGFAPCre-induced ZsGreen Cre reporter fluorescence in extrahepatic bile ducts, the brain and brain sections ( n =1). ( b , c ) HSCs were isolated from hGFAPCre mice expressing ZsGreen ( n =2) and were either plated ( b ) or analysed by flow cytometry ( c ). LratCre mice served as positive control ( n =3). ( d ) HSCs were isolated from hGFAPCre mice expressing mTom/mGFP Cre reporter and plated ( n =1). ( e ) Sections from untreated ( n =1), bile duct-ligated ( n =1) and CCl 4 -treated livers ( n =2) were stained for desmin, showing no co-localization of ZsGreen and HSC marker desmin by confocal microscopy. ( f ) Representative western blotting (out of n =3) showing cytokeratin 19 expression but no desmin expression in fluorescence-activated cell sorting-sorted hGFAPCre-labelled ZsGreen-positive cells. ( g ) hGFAPCre mice undergoing either BDL ( n =1) or CCl 4 treatment ( n =1) show no overlap between tdTomato Cre reporter and Col-GFP reporter, thus excluding a contribution of hGFAPCre-labelled cells to ECM-producing myofibroblasts. ( h ) Cytokeratin staining of bile duct-ligated hGFAPCre mice shows almost complete overlap of cytokeratin, marking the bile duct proliferates, and hGFAPCre-induced ZsGreen expression ( n =1). ( i ) Sections from untreated mice expressing Cre under the murine Gfap promoter and mTom/mGFP Cre reporter show no GFP expression in the liver. The brain served as the positive control (Inlet). Scale bars, 4 mm ( a , left panel), 2 mm ( a , upper middle and right panel), 200 μm ( a , lower middle and right panel) and 50 μm ( b , d , e , g – i ). 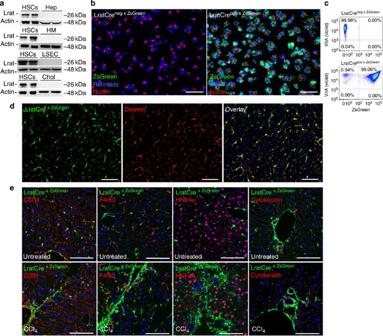Figure 2: LratCre efficiently labels HSCs. (a) Lrat expression was determined by western blotting in pure and never-plated primary murine HSCs (n=8), hepatocytes (n=2), Kupffer cells (n=2), endothelial cells (n=2) and cholangiocytes (n=2). (b,c) HSCs were isolated from LratCre-negative (n=2) and LratCre-positive mice (n=3) expressing ZsGreen Cre reporter and were either plated for 24 h (b) or analysed by flow cytometry (c), using vitamin A (‘VitA’, determined in the violet fluorescence-activated cell sorting channel) fluorescence as HSC marker in both approaches. (d) Co-localization of LratCre-induced ZsGreen expression and desmin was determined in untreated livers using confocal microscopy (n=4). (e) Co-localization of LratCre-induced ZsGreen expression and CD31 (marking endothelial cells), F4/80 (marking macrophages), HNF4α (marking hepatocytes) and cytokeratin (marking cholangiocytes) was determined by confocal microscopy in untreated and CCl4-treated mice. Scale bars, 100 μm (b,d,e). Full size image Figure 2: LratCre efficiently labels HSCs. ( a ) Lrat expression was determined by western blotting in pure and never-plated primary murine HSCs ( n =8), hepatocytes ( n =2), Kupffer cells ( n =2), endothelial cells ( n =2) and cholangiocytes ( n =2). ( b , c ) HSCs were isolated from LratCre-negative ( n =2) and LratCre-positive mice ( n =3) expressing ZsGreen Cre reporter and were either plated for 24 h ( b ) or analysed by flow cytometry ( c ), using vitamin A (‘VitA’, determined in the violet fluorescence-activated cell sorting channel) fluorescence as HSC marker in both approaches. ( d ) Co-localization of LratCre-induced ZsGreen expression and desmin was determined in untreated livers using confocal microscopy ( n =4). ( e ) Co-localization of LratCre-induced ZsGreen expression and CD31 (marking endothelial cells), F4/80 (marking macrophages), HNF4α (marking hepatocytes) and cytokeratin (marking cholangiocytes) was determined by confocal microscopy in untreated and CCl 4 -treated mice. Scale bars, 100 μm ( b , d , e ). Full size image HSCs are the main contributors to toxic liver fibrosis To determine the contribution of HSCs to the myofibroblast pool, we first subjected LratCre mice to the well-established model of carbon tetrachloride (CCl 4 )-induced liver fibrosis. In this model, LratCre-induced ZsGreen expression—marking HSCs—and α-smooth muscle actin (αSMA) expression—marking myofibroblasts—completely overlapped, and displayed micro- and macroscopic ZsGreen fluorescence with the characteristic septal pattern of liver fibrosis ( Fig. 3a,b ). To determine the relative contribution of HSCs to the myofibroblast pool, we quantified the overlap between LratCre-induced Cre reporter and αSMA. In CCl 4 -induced liver fibrosis, the overlap between LratCre-induced ZsGreen and αSMA was 93.6% (±2.3% s.d., n =4, Fig. 3b ), providing evidence that HSCs are the almost exclusive source of myofibroblasts in toxic liver fibrosis. To confirm this data by a second approach, we generated LratCre mice co-expressing red-fluorescent Cre reporter tdTomato and a green-fluorescent Col-GFP reporter, which faithfully marks collagen-producing cells [22] . LratCre-induced tdTomato almost completely overlapped with Col-GFP fluorescence in the CCl 4 model (96.0%±2.4% s.d., n =4, Fig. 3b ), thus matching the degree of overlap that we found between αSMA and LratCre-induced ZsGreen. Accordingly, nearly all αSMA-positive cells were also Col-GFP-positive ( Fig. 3c ). To exclude that our data may be specific to the CCl 4 model, we confirmed our findings in a second well-established model of toxic liver fibrosis, induced by thioacetamide (TAA) treatment. Livers from TAA-induced treated mice also displayed a characteristic macro- and microscopic septal pattern of ZsGreen fluorescence, and the same range of co-localization between LratCre-induced TdTomato and Col-GFP fluorescence (94.8±0.3% s.d., n =3) as in the CCl 4 model ( Supplementary Fig. S2A–C ). To further substantiate the functional contribution of HSCs to fibrogenesis, we ablated HSCs via LratCre-induced diphtheria toxin receptor. This strategy strongly reduced HSC numbers in untreated and CCl 4 -treated livers, albeit not completely ( Fig. 3d,e and Supplementary Fig. S3A ). However, it should be noted that this approach typically does not result in complete ablation unless a strongly intensified regimen of diptheria toxin injection is employed [23] . The reduction of αSMA and profibrogenic gene expression by at least the same degree as ablation of HSCs, assessed by desmin mRNA and immunohistochemisty ( Fig. 3d,e ), confirms the relevant contribution of HSCs to fibrogenesis. In contrast, hepatic inflammation, injury and expression of endothelial marker vWf were not affected by HSC ablation ( Supplementary Fig. S3B–D ). 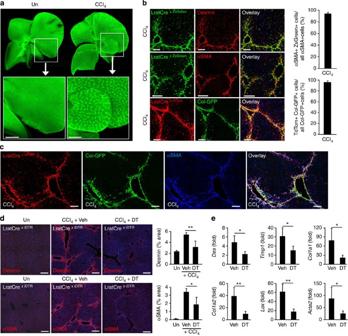Figure 3: HSCs are the principal source of myofibroblasts in CCl4-induced liver fibrosis. (a) Representative fluorescent images of whole livers from untreated and CCl4-treated mice (n=3) show LratCre-labelled ZsGreen-positive macroscopic fibrotic septa in CCl4-treated liver. (b). Frozen liver sections from CCl4-treated LratCre-positive mice were stained with desmin (upper panel) or αSMA (middle panel) to demonstrate co-localization of HSC marker desmin or αSMA and LratCre-induced ZsGreen by confocal microscopy. Confocal microscopy was employed to show co-localization of Col-GFP reporter, marking activated myofibroblasts and LratCre-induced tdTomato expression (lower panel). Quantification of αSMA-expressing cells that are derived from LratCre-labelled ZsGreen-positive HSCs in fibrosis induced by 9 × CCl4(n=4, upper graph) or Col-GFP-expressing cells that are derived from LratCre-labelled tdTomato-positive HSCs in fibrosis induced by 9 × CCl4treatment (n=4, lower graph). (c) Co-localization of αSMA with tdTomato and Col-GFP in 9 × CCl4-induced liver fibrosis was determined by confocal microscopy employing far-red secondary antibody for αSMA detection. (d,e) LratCre mice, expressing Cre-inducible diphteria toxin receptor (iDTR) received either vehicle (n=4) or dipheria toxin (DT,n=4) during CCl4-induced liver fibrosis induction. Expression of αSMA and desmin was determined by immunohistochemstry and quantified (d), expression of fibrogenic genes was determined by qPCR (e). Scale bars, 1 mm (a), 100 μm (b,c) and 200 μm (d). Data are shown as means±s.d. *P<0.05, **P<0.01 (determined by Student’st-test). Figure 3: HSCs are the principal source of myofibroblasts in CCl 4 -induced liver fibrosis. ( a ) Representative fluorescent images of whole livers from untreated and CCl 4 -treated mice ( n =3) show LratCre-labelled ZsGreen-positive macroscopic fibrotic septa in CCl 4 -treated liver. ( b ). Frozen liver sections from CCl 4 -treated LratCre-positive mice were stained with desmin (upper panel) or αSMA (middle panel) to demonstrate co-localization of HSC marker desmin or αSMA and LratCre-induced ZsGreen by confocal microscopy. Confocal microscopy was employed to show co-localization of Col-GFP reporter, marking activated myofibroblasts and LratCre-induced tdTomato expression (lower panel). Quantification of αSMA-expressing cells that are derived from LratCre-labelled ZsGreen-positive HSCs in fibrosis induced by 9 × CCl 4 ( n =4, upper graph) or Col-GFP-expressing cells that are derived from LratCre-labelled tdTomato-positive HSCs in fibrosis induced by 9 × CCl 4 treatment ( n =4, lower graph). ( c ) Co-localization of αSMA with tdTomato and Col-GFP in 9 × CCl 4 -induced liver fibrosis was determined by confocal microscopy employing far-red secondary antibody for αSMA detection. ( d , e ) LratCre mice, expressing Cre-inducible diphteria toxin receptor (iDTR) received either vehicle ( n =4) or dipheria toxin (DT, n =4) during CCl 4 -induced liver fibrosis induction. Expression of αSMA and desmin was determined by immunohistochemstry and quantified ( d ), expression of fibrogenic genes was determined by qPCR ( e ). Scale bars, 1 mm ( a ), 100 μm ( b , c ) and 200 μm ( d ). Data are shown as means±s.d. * P <0.05, ** P <0.01 (determined by Student’s t -test). Full size image HSCs are the main contributors to biliary liver fibrosis After having established HSCs as the main contributors to toxic liver fibrosis, we next determined the contribution of HSCs to cholestatis-induced liver fibrosis. In this setting, portal fibroblasts are believed to be an essential contributor to fibrogenesis [4] , [5] , [7] . In three well-established models of cholestasis-induced liver fibrosis, bile duct ligation (BDL), 3,5-diethoxycarbonyl-1,4-dihydro-collidine (DDC)-containing diet and Mdr2 ko mice, tdTomato expression almost completely overlapped with Col-GFP reporter expression, reaching 89% co-localization and thus almost the same degree as in toxic liver fibrosis ( Fig. 4a–c,e ). This data was confirmed by flow cytometric analysis of the entire non-parenchymal cell pool, in which 82–85% of collagen-producing cells were tdTomato-positive HSCs ( Fig. 4d,e ). A high contribution of HSCs to collagen-producing cells was even noted during early cholestatic liver fibrosis (87–90% co-localization, Supplementary Fig. S4A–D, G ) and in the methionine–choline-deficient diet model of non-alcoholic steatohepatitis ( Supplementary Fig. S4E–G ). Similar to CCl 4 -induced liver fibrosis, LratCre not only marked collagen-producing cells but also αSMA-expressing cells, with 80 and 88% overlap between αSMA and LratCre-induced tdTomato after 7 and 14 days BDL, respectively, and a strong overlap between αSMA-positive and Col-GFP-positive cells ( Supplementary Fig. S5A,B ). 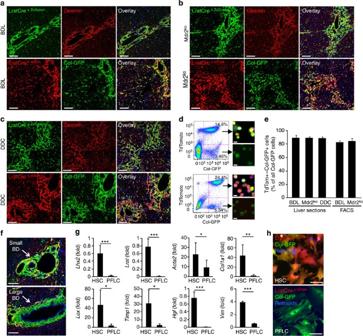Figure 4: HSCs are the principal source of myofibroblasts in cholestatic liver fibrosis. (a–c) Liver sections of 14 day bile duct-ligated (BDL) mice (a, ZsGreenn=3, tdTom/Col-GFPn=4), 9-week-old Mdr2komice (b, ZsGreenn=4, tdTom/Col-GFPn=5), or 0.1% DDC-diet-treated mice (c, ZsGreenn=4, tdTom/Col-GFPn=3) were stained with desmin to demonstrate co-localization of HSC marker desmin and LratCre-induced ZsGreen by confocal microscopy (upper panel). Confocal microscopy was employed to show co-localization of Col-GFP reporter, marking activated myofibroblasts and LratCre-induced tdTomato expression (lower panel). (d) Flow cytometric images from 2-week-old BDL mice (upper panel) and 9-week-old Mdr2ko(lower panel) mice co-expressing LratCre, tdTomato and Col-GFP. Images next to fluorescence-activated cell sorting (FACS) plots show sorted cells freshly after plating. (e) Quantification of Col-GFP-expressing cells, derived from LratCre-labelled tdTomato-positive HSCs, was performed in liver sections (14 days BDL:n=4; Mdr2kon=5; 0.1% DDC diet:n=3) or in non-parenchymal cell fractions using flow cytometry (14 days BDL:n=4, Mdr2kon=6). (f) Images demonstrating small and large bile ducts surrounded by Col-GFP-positive and LratCre-negative portal fibroblasts. (g) Quantitative PCR analysis of FACS-sorted unplated LratCre-labelled tdTom-positive and Col-GFP-positive cells (HSC,n=5 isolates), and tdTom-negative and Col-GFP-positive cells (PFLCs,n=5 isolates). (h) Representative images of HSCs and PFLCs show morphologically distinct cell populations. Scale bars, 100 μm (a–c), 10 μm (d), 100 μm (f) and 50 μm (h). Data are shown as means±s.d. *P<0.05; **P<0.01; ***P<0.001 (determined by Student’st-test). Figure 4: HSCs are the principal source of myofibroblasts in cholestatic liver fibrosis. ( a – c ) Liver sections of 14 day bile duct-ligated (BDL) mice ( a , ZsGreen n =3, tdTom/Col-GFP n =4), 9-week-old Mdr2 ko mice ( b , ZsGreen n =4, tdTom/Col-GFP n =5), or 0.1% DDC-diet-treated mice ( c , ZsGreen n =4, tdTom/Col-GFP n =3) were stained with desmin to demonstrate co-localization of HSC marker desmin and LratCre-induced ZsGreen by confocal microscopy (upper panel). Confocal microscopy was employed to show co-localization of Col-GFP reporter, marking activated myofibroblasts and LratCre-induced tdTomato expression (lower panel). ( d ) Flow cytometric images from 2-week-old BDL mice (upper panel) and 9-week-old Mdr2 ko (lower panel) mice co-expressing LratCre, tdTomato and Col-GFP. Images next to fluorescence-activated cell sorting (FACS) plots show sorted cells freshly after plating. ( e ) Quantification of Col-GFP-expressing cells, derived from LratCre-labelled tdTomato-positive HSCs, was performed in liver sections (14 days BDL: n =4; Mdr2 ko n =5; 0.1% DDC diet: n =3) or in non-parenchymal cell fractions using flow cytometry (14 days BDL: n =4, Mdr2 ko n =6). ( f ) Images demonstrating small and large bile ducts surrounded by Col-GFP-positive and LratCre-negative portal fibroblasts. ( g ) Quantitative PCR analysis of FACS-sorted unplated LratCre-labelled tdTom-positive and Col-GFP-positive cells (HSC, n =5 isolates), and tdTom-negative and Col-GFP-positive cells (PFLCs, n =5 isolates). ( h ) Representative images of HSCs and PFLCs show morphologically distinct cell populations. Scale bars, 100 μm ( a – c ), 10 μm ( d ), 100 μm ( f ) and 50 μm ( h ). Data are shown as means±s.d. * P <0.05; ** P <0.01; *** P <0.001 (determined by Student’s t -test). Full size image Lrat-negative portal fibroblasts-like cells are distinct from HSCs In addition to LratCre-labelled, Col-GFP-positive HSCs, we also found a small population of Col-GFP-positive but LratCre-unlabelled fibroblasts, both in the liver and in cell isolates of cholestatic fibrosis models. These cells were predominantly located around the portal tracts and did not contain retinoid lipid droplets, consistent with characteristics of portal fibroblasts ( Fig. 4f,h ). This LratCre-negative, Col-GFP-positive population of portal fibroblast-like cells (PFLCs) showed low expression of genes characteristic for HSCs, such as Lrat , Lhx2 and HGF , and was morphologically distinct from HSCs ( Fig. 4g,h ). PFLCs were αSMA- and Col-GFP-positive, and abundantly expressed Acta2 , Col1a1 , Lox , Timp1 and Vim in comparison with whole liver ( Supplementary Fig. S6A,B ), confirming them as myofibroblasts. However, they expressed significantly lower levels of fibrogenic genes than HSCs in our isolates ( Fig. 4g ), thus excluding that PFLC might represent a less abundant but more fibrogenic population than HSCs. Together, these data indicate that portal fibroblast constitute a myofibroblast population that is not HSC-derived and significantly less abundant than HSCs, and probably fulfils specialized functions in cholestatic liver disease. Myofibroblasts derive from LratCre-labelled retinoid-positive HSCs αSMA staining in normal liver (where HSCs are quiescent and do not express αSMA) revealed that LratCre also labelled some vascular smooth muscle cells (VSMCs, Supplementary Fig. S7A ). This may be explained by the fact that VSMCs and pericytes/HSCs are considered to be of the same lineage [24] , sharing a common precursor in the liver [25] . Although LratCre-labelled HSCs outnumbered LratCre-labelled VSMCs by a factor of >200 ( Supplementary Fig. S7B ), we wanted to further exclude a major contribution of LratCre-labelled VSMCs, or any other non-HSC population to the hepatic collagen-producing fibroblast pool. As specific labelling of hepatic VSMCs is not feasible, we employed retinoid fluorescence to identify LratCre-labelled myofibroblasts of HSC origin. Retinoid fluorescence was observed in >90% of tdTomato- and Col-GFP-positive cells in the CCl 4 , BDL and Mdr2 ko fibrosis models ( Supplementary Fig. S7C,D ), albeit at a lower level than in quiescent HSCs, thus confirming that these myofibroblasts are of HSC and not of VSMC origin. Collectively, our data establish HSCs as principal contributors to the collagen-producing myofibroblast pool across all types of liver fibrosis. HSCs are not epithelial progenitors Next, we determined whether HSCs may exert functions besides fibrogenesis in liver injury. Previous studies, employing hGFAPCre and αSMA-CreERT2 mice for fate tracing, suggested that up to 24% of hepatocytes were derived from HSCs in the methionine–choline-deficient ethionine-supplemented (MCDE) diet and BDL models [18] , [19] . By employing LratCre mice, we tested whether short- and long-term injury induced by BDL, Mdr2 ko , MCDE diet, DDC diet, CCl 4 , TAA or 70% partial hepatectomy resulted in the generation of HNF4α-positive hepatocytes expressing ZsGreen Cre reporter, thus identifying them as progeny of LratCre-expressing HSCs. Although we found rare HNF4α-positive hepatocytes (at a frequency of ≈0.2 per 1,000 cells) expressing Cre reporter ZsGreen, none of the injury models increased this rate in the liver ( Fig. 5a–g and Supplementary Fig. S8A–C ). We also did not observe increased ZsGreen-positive cells with hepatocyte morphology (positive control shown in the insert of Fig.5A) in liver sections ( Fig. 5a–f and Supplementary Fig. S8B–C ) or in primary hepatocyte isolates ( Fig. 5h,i and Supplementary Fig. S8D ). Furthermore, LratCre-marked cells did not give rise to cytokeratin-positive liver progenitor cells or cholangiocytes in any of the chronic injury models ( Fig. 2e and Supplementary Fig. S9A–E ). Collectively, these data exclude that HSCs function as epithelial progenitors. 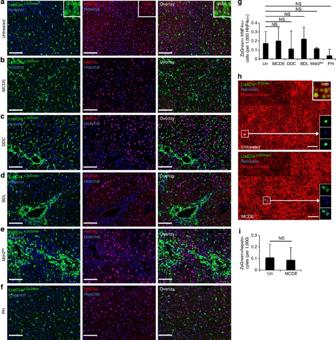Figure 5: HSCs do not contribute to the generation of newly formed hepatocytes. (a–g) Determination of possible co-localization of hepatocyte marker HNF4α and LratCre-induced ZsGreen was performed by confocal microscopy in untreated mice (n=4;a), mice receiving MCDE diet for 3 weeks followed by 3 weeks recovery on regular chow (n=4;b), mice receiving DDC diet for 4 weeks followed by 3 weeks recovery (n=3;c), mice undergoing BDL for 2 weeks (n=3;d), 9- to 15-week-old Mdr2ko mice (n=3;e), or 2 weeks after partial hepatectomy (n=3;f). The number of HNF4α-expressing hepatocytes, positive for ZsGreen, was quantified from confocal microscope images (g). (h,i) Representative images of primary hepatocytes isolated from control mice (n=3) and mice that received MCDE diet for 3 weeks (n=4), followed by 3 weeks recovery (h). Positive control (‘+ ctrl’) from AAV8-TBG-Cre-injected mice showing ZsGreen-positive hepatocytes (n=1;h, upper right insert). The rare ZsGreen-positive small-size cells were identified as HSCs by their characteristic fluorescent retinoid-containing lipid droplets (h, lower right inserts). ZsGreen-positive hepatocytes were quantified (i). Scale bar, 100 μm. Data are shown as means±s.d.; NS, non-significant (one-way analysis of variance). Figure 5: HSCs do not contribute to the generation of newly formed hepatocytes. ( a – g ) Determination of possible co-localization of hepatocyte marker HNF4α and LratCre-induced ZsGreen was performed by confocal microscopy in untreated mice ( n =4; a ), mice receiving MCDE diet for 3 weeks followed by 3 weeks recovery on regular chow ( n =4; b ), mice receiving DDC diet for 4 weeks followed by 3 weeks recovery ( n =3; c ), mice undergoing BDL for 2 weeks ( n =3; d ), 9- to 15-week-old Mdr2ko mice ( n =3; e ), or 2 weeks after partial hepatectomy ( n =3; f ). The number of HNF4α-expressing hepatocytes, positive for ZsGreen, was quantified from confocal microscope images ( g ). ( h , i ) Representative images of primary hepatocytes isolated from control mice ( n =3) and mice that received MCDE diet for 3 weeks ( n =4), followed by 3 weeks recovery ( h ). Positive control (‘+ ctrl’) from AAV8-TBG-Cre-injected mice showing ZsGreen-positive hepatocytes ( n =1; h , upper right insert). The rare ZsGreen-positive small-size cells were identified as HSCs by their characteristic fluorescent retinoid-containing lipid droplets ( h , lower right inserts). ZsGreen-positive hepatocytes were quantified ( i ). Scale bar, 100 μm. Data are shown as means±s.d. ; NS, non-significant (one-way analysis of variance). Full size image LratCre-positive HSCs are not BM derived Finally, we employed LratCre mice to assess whether HSCs constitute a liver-resident or BM-derived cell population, a point of substantial controversy [26] , [27] , [28] . We did not detect LratCre-labelled HSCs in normal liver or fibrotic livers after BDL or long-term injury induced by 20 CCl 4 injections despite successful BM transplantation as evidenced by mTom-positive (that is, non-recombined) BM-derived cells in the spleen and mTom- and F4/80-double-positive BM-derived macrophages in the liver ( Fig. 6a–c ). These data confirm HSCs as liver-resident cell population. 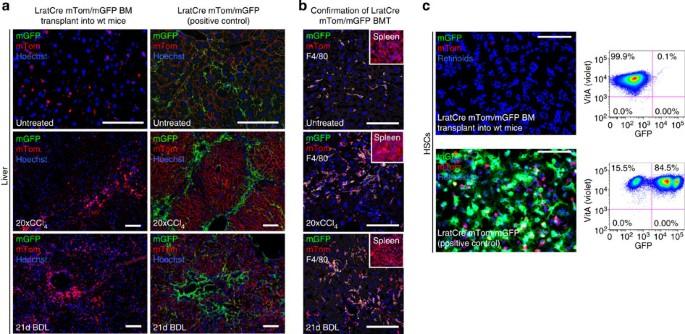Figure 6: LratCre-labelled HSCs are not BM-derived. (a–c) BM from mice expressing LratCre and mTom/mGFP Cre reporter was transplanted into lethally irradiated wild-type recipients. Untreated (n=2), 20 × CCl4(n=1) and 3 weeks BDL (n=1) treated mice were killed 5–6 months after BM transplantation and showed no LratCre-induced mGFP expression, thus excluding a contribution of the BM to generation of LratCre-expressing HSCs. In contrast, LratCre-positive mice expressing mTom/mGFP, serving as positive control, showed abundant mGFP signal (a). Successful BMT was confirmed by the presence mTom-positive cells in the spleen (see inserts) and demonstration of F4/80-positive mGFP-expressing liver macrophages (b). HSCs isolated from BM-transplanted mice (n=1) showed no mGFP signal or by flow cytometric analysis, whereas controls showed abundant mGFP signal (n=4;c). Scale bar, 100 μm. Figure 6: LratCre-labelled HSCs are not BM-derived. ( a – c ) BM from mice expressing LratCre and mTom/mGFP Cre reporter was transplanted into lethally irradiated wild-type recipients. Untreated ( n =2), 20 × CCl 4 ( n =1) and 3 weeks BDL ( n =1) treated mice were killed 5–6 months after BM transplantation and showed no LratCre-induced mGFP expression, thus excluding a contribution of the BM to generation of LratCre-expressing HSCs. In contrast, LratCre-positive mice expressing mTom/mGFP, serving as positive control, showed abundant mGFP signal ( a ). Successful BMT was confirmed by the presence mTom-positive cells in the spleen (see inserts) and demonstration of F4/80-positive mGFP-expressing liver macrophages ( b ). HSCs isolated from BM-transplanted mice ( n =1) showed no mGFP signal or by flow cytometric analysis, whereas controls showed abundant mGFP signal ( n =4; c ). Scale bar, 100 μm. Full size image Despite the lack of solid in vivo evidence that HSCs are the primary drivers of liver fibrosis, much of the current research and drug discovery work focus on this cell type. After the discovery that HSCs produce significantly larger amounts of collagen than hepatocytes and endothelial cells in vitro and thus constitute a prime candidate for hepatic myofibroblast precursors [11] , little progress has been made to further establish and precisely quantify the relative contribution of HSCs to the hepatic myofibroblast pool and liver fibrosis in vivo . Most subsequent studies have investigated HSC activation in cell cultures, a process that differs substantially from in vivo activation [10] , [29] , or studied HSC isolates from normal and fibrotic livers [10] , [12] . Because of the lack of fate tracing techniques that specifically label precursor populations such as HSCs, sources of hepatic myofibroblasts have not yet been established or precisely quantified in vivo . Fate tracing has excluded a contribution for epithelial cells to the hepatic myofibroblast pool [13] , [14] , [15] and characterized the embryonic origin of HSCs [16] . However, positive identification of myofibroblast precursors has not been achieved, as fate-tracing approaches have labelled all myofibroblast populations but not specific precursors [13] or subpopulations, such as subcapsular fibroblasts, which contribute little to organ fibrosis and the deleterious complications of fibrosis due to their sparsity and anatomic location [16] . The most important finding of our study is the in vivo identification of HSCs as a universal and liver-resident source for myofibroblasts, exerting a dominant role across toxic, biliary and fatty liver diseases. These data suggest that HSCs should be considered the primary target for the development of new antifibrotic therapies, which has become an important focus of the field [30] , [31] , [32] . Revealing HSCs as the by-far dominant source in cholestatic fibrosis is unexpected, as portal fibroblasts have been considered a key contributor in cholestatic liver fibrosis [4] , [5] , [7] . The consistently high contribution of HSCs was observed in three different models of cholestasis, including the Mdr2 ko model, which mimicks defects in cholestatic patients [33] . Thus, our data refute the hypothesis that the underlying disease dictates the cell type that contributes to the myofibroblast pool in liver fibrosis, and instead establish HSCs as universal responders that trigger wound repair across different types of liver injury. Despite the dominant role of HSCs, there was a higher contribution of non-HSC myofibroblast sources in biliary than in toxic liver fibrosis. Accordingly, we identified a population of LratCre-negative fibroblasts around portal tracts that were distinct from HSCs in terms of gene expression and anatomic localization. Despite being less abundant than HSCs, these cells most likely exert important functions in cholestatic liver disease. Although portal fibroblasts probably do not make a major contribution to organ fibrosis and associated complications such as portal hypertension owing to their low abundance, their anatomic localization suggests that they may exert specialized functions related to bile ducts. This might be the mechanical stabilization of bile ducts as an adaptive response to increased pressure, or a contribution to biliary stenosis as a maladaptive response. It is also conceivable that portal fibroblasts represent a cell population that has a role in early biliary fibrosis serving as ‘rapid responders’ [7] , and that it is essential in recruiting HSCs, which then in turn contribute to the majority of ECM production. Further studies should also determine whether LratCre-negative portal fibroblasts may produce different type of ECM than HSCs. The second relevant finding of our study is that HSCs are not progenitor cells and do not contribute to the generation of hepatocytes in the injured liver. Previous studies had suggested that HSCs contribute up to 24% of newly formed hepatocytes [18] , [19] . As we labelled >99% of HSCs by LratCre and investigated their contribution to hepatocyte generation in liver sections from seven different injury models and in primary hepatocyte isolates from two injury models, in the liver and in hepatocyte isolates without finding increased number of HNF4α- and ZsGreen-double positive cells, or ZsGreen-positive cells with hepatocyte shape, we can exclude HSCs as a source for epithelial regeneration in the liver. Our findings are congruent with studies showing that hepatocytes and, to a lesser degree, bipotential progenitors function as efficient cellular sources for epithelial regeneration [34] , [35] , [36] . Finally, our data, showing that GFAPCre transgenic mice efficiently label cholangiocytes but not a significant amount of HSCs, suggest that previous studies employing GFAPCre [13] , [18] , [19] , [37] , [38] are likely to be not HSC-specific. We cannot completely rule out that there may be differences in the recombination in different floxed alleles or Cre reporters, but have tested three Cre reporters, confirmed GFAPCre by sequencing, tested functional Cre expression in brain sections and have used mice expressing Cre under the human GFAP as well as the murine Gfap promoter. Furthermore, previous publications [18] , [19] and Jackson Laboratories ( https://ndp.jax.org/NDPServe.dll?ViewItem?ItemID=1741&XPos=11536496&YPos=5169511&ZPos=0&Lens=1.25&SignIn=Sign%20in%20as%20Guest ) have reported Cre activity in cholangiocytes. Our study has several limitations. First of all, murine fibrogenesis may not fully reflect human fibrogenesis due to its shorter duration, different biology and difficulties to model all relevant diseases adequately in mice. We have assessed the HSC contribution in a large number of murine models, but human confirmation is warranted. This may be achieved by developing markers that clearly distinguish between HSC and non-HSC myofibroblast populations such as portal fibroblasts. Second of all, LratCre also labelled some VSMCs in our study. This is likely to be because of the fact that pericytes and VSMCs share a common precursor in many organs, including the liver [24] , [25] . However, we found that >90% of LratCre-labelled myofibroblasts contained retinoid lipid droplets characteristic for HSCs, thus providing strong evidence that LratCre-labelled myofibroblasts are indeed derived from HSCs. Third, it is conceivable that LratCre activity is turned on in non-HSC populations during fibrogenesis, and that we overestimate the contribution of HSCs. However, we found that non-HSC myofiboblast populations such as PFLCs were LratCre-negative and distinct from HSC. We also did not find a significant amount of LratCre-labelled hepatocytes, cholangiocytes, endothelial cells or Kupffer cells in CCl 4 -induced liver injury, providing further evidence that LratCre activity is not significantly induced in non-HSC populations in the injured liver. Moreover, the above discussed finding that >90% of LratCre-positive myofibroblasts also contained retinoids characteristic for HSCs also excludes a significant contribution of non-HSC populations. As such, retinoid lipid droplets are a defining feature of HSCs and the only parameter by which they could be clearly defined to date. Tamoxifen-inducible LratCre would be helpful to further confirm these data and further exclude LratCre activity in other cell types during disease, but is likely to achieve a lower labelling efficacy than constitutive LratCre and a less precise quantification of HSC contribution to the hepatic myofibroblast pool. Fourth, our isolation of PFLCs may contain cells other than portal fiboblasts as the employed isolation method relied on exclusion of HSCs and not on positive identification. Further establishment of high purity portal fibroblast isolates will allow more powerful qualitative comparison between HSCs and portal fibroblasts. In contrast to the dominant role of HSCs in liver fibrosis, the contribution of pericytes in fibrosis of other organs remains controversial with some studies in the kidney, lung and spinal cord [39] , [40] , [41] showing a key contribution but other studies reporting opposite findings [42] , [43] . Confirming a key role for pericytes in fibrogenesis in additional organs may allow to determine common targets for antifibrotic therapies across different organs. Generation of LratCre mice A Cre-containing cassette was PCR-amplified with 60-bp overhangs homologous to the upstream and downstream sequence surrounding the ATG site of the mouse Lrat gene. The PCR product was inserted into a BAC containing the mouse Lrat gene by recombineering. After removal of the Neo cassette by arabinose-induced flippase, BAC DNA was microinjected into the pronucleus of fertilized CBAxC57BL/6J oocytes. Out of six positive founders, the one showing the strongest LratCre-induced Cre reporter expression in the liver and HSCs was used for further studies. Pups were born in a male/female ratio of 1:1 (50.3% versus 49.7%, n =179). Mice and genotyping Mice in which Cre expression is driven by the human GFAP promoter (hGFAPCre) [44] , the murine Gfap promoter (mGfapCre) [45] and mice expressing Cre reporters ZsGreen, TdTomato [46] or mTom/mGFP [47] were obtained from Jackson. Mdr2ko mice [48] in FVB/N background have been described. For all experiments, LratCre mice were maintained in a mixed background after breeding one to two times into the ZsGreen, tdTomato reporter and mTom/mGFP strains of the C57Bl/6 background, or Mdr2ko mice. Mice for HSC isolations were used at ages 12–18 weeks. Mice used for fibrosis or injury models, or for non-parenchymal cell isolation were used at ages 8–12 weeks unless otherwise indicated. Mice of both genders were used with the exception of the BDL and DDC models for which only male mice were employed. Genotyping for LratCre was done using forward primer 5′-CCTTTCTTTGACCCCCTGCAC-3′ and reverse primer 5′-GACCGGCAAACGGACAGAAG-3′. Genotyping for hGFAPCre mice was done using forward primer 5′-ACTCCTTCATAAAGCCCT-3′ and reverse primer 5′-CGCCGCATAACCAGTGAAAC-3′. The PCR product for hGFAPCre genotyping was sequenced and presence of human GFAP promoter sequence was confirmed. Liver fibrosis and injury models Toxic liver fibrosis was induced by intraperitoneal injections of either CCl 4 (0.5 μl g −1 , dissolved in corn oil at a ratio of 1:3) for various intervals, or of TAA (dissolved in NaCl 0.9%) for 6 weeks (three injections per week) at increasing concentrations (first dose: 50 mg kg −1 , second dose: 100 mg kg −1 , third to sixth dose: 200 mg kg −1 , all following doses: 300 mg kg −1 ) as previously described [49] . For the induction of cholestatic liver fibrosis, mice underwent ligation of the common bile duct [27] . Briefly, after abdominal incision, the common bile duct was ligated distally. For additional models of cholestatic liver fibrosis, mice were either fed a 0.1% DDC-containing diet for 4 weeks or LratCre mice were crossed with Mdr2ko mice [48] in FVB/N background. ZsGreen, tdTomato and mTom/mGFP Cre reporter mice [46] , [47] , as well as Col-GFP reporter [22] mice, have been described elsewhere. As a model of fatty liver disease, liver fibrosis was induced by feeding mice a methione–choline-deficient diet for 9 weeks. Seventy per cent partial hepatectomy was performed as described [50] . Briefly, after midline abdominal incision, the left lateral and the median liver lobes were mobilized, ligated and cut off [50] . As models of liver injury with progenitor expansion, we employed the above described DDC diet and methionine–choline-deficient diet combined with 0.15% ethionine supplementation in drinking water (MCDE diet) [18] , [19] . All animal procedures were in accordance with guidelines by the National Institutes of Health and were approved by the Institutional Animal Care and Use Committee at Columbia University. Primary cell isolations HSCs were isolated from mice as described previously [49] , [51] . Briefly, after cannulation of the inferior vena cava, the portal vein was cut, allowing retrograde stepwise perfusion with pronase (Sigma-Aldrich, St Louis, MO, USA)- and collagenase (Roche, Germany)-containing solutions, and subsequent 9.7% Nycodenz gradient centrifugation. Purity was assessed by vitamin A autofluorescence under a fluorescent microscope (Olympus 71IX). The entire population of non-parenchymal cells was isolated using pronase/collagenase perfusion and a 16.95% Nycodenz gradient. Murine hepatocytes were isolated by collagenase perfusion and low-density centrifugation with Percoll [52] . F4/80-positive hepatic macrophages were isolated after collagenase/pronase perfusion, followed by a 16.95% Nycodenz gradient and subsequent positive selection of F4/80-positive cells by magnetic-activated cell sorting (MACS) using biotinylated F4/80 antibody (clone: BM8; eBioscience, San Diego, CA, USA) and anti-biotin MACS beads (Miltenyi Biotec, Auburn, CA, USA) [53] . On the basis of the specific marking of bile ducts by hGFAPCre, cholangiocytes were isolated by flow cytometry from hGFAPCre mice expressing ZsGreen Cre reporter after pronase/collagenase perfusion of mouse livers. Cholangiocyte identity was confirmed by western blotting for cytokeratin 19. Liver sinusoidal endothelial cells were isolated by collagenase perfusion followed by MACS using anti-CD146 MACS beads (Miltenyi Biotec) and subsequent FACS analysis to exclude HSCs in the isolate [54] . Analysis of vitamin A content and Col-GFP expression Vitamin A fluorescence was analysed by flow cytometry in isolated HSCs or non-parenchymal liver cells using 405–407 nm lasers for excitation and a 450/50-nm bandpass filter for detection. To determine vitamin A expression of activated HSCs, Col-GFP- and tdTomato-double-positive cells were gated. Vitamin A-negative cells expressing Col-GFP were used as negative controls to set the threshold for positive signals for Vitamin A. GFP expression was analysed using 488 nm lasers and 530/30 nm bandpass filter for detection. Non-parenchymal liver cell isolations from untreated Col-GFP-positive, LratCre-positive and tdTomoto-positive mice were used to set the threshold for positive Col-GFP signals. TdTomato expression was analysed using 488 nm lasers and 582/15 nm bandpass filter for detection. Four to six independent cell isolates were analysed for each model, using a minimum for 100,000 events for data evaluation. Flow cytometric data were analysed by FlowJo software. BM transplantation BM transplantation was performed as described previously [27] . Briefly, wild-type mice were macrophage depleted by injection of liposomal clodronate, followed by lethal irradiation with 2 × 6 Gy and intravenous injection of 10 × 10 6 BM cells from LratCre-positive, mTom/mGFP mice. Successful BM transplantation was confirmed by the presence of mTom-positive cells in the spleen and mTom-positive macrophages in the liver. Immunohistochemical staining and microscopy Immunohistochemistry was performed on frozen liver sections. Mouse livers were perfused with 4% paraformaldehyde and embedded. Frozen tissue blocks were cut to yield 5 μm sections for immunohistochemical staining [49] using primary antibodies against desmin (1:300, rabbit, Lab Vision catalogue number RB-9014-P; Thermo Fisher Scientific, Fremont, CA, USA), αSMA (1:500, mouse, fluorescein isothiocyanate-conjugated, Sigma-Aldrich F3777), cytokeratin (1:250, rabbit, DAKO Z0622), F4/80 (1:250, rat, AbD serotec MCA497A64), CD31 (1:500, rat, Pharmingen 553369), PDGFRβ (1:50, rabbit, Cell Signaling 3169) and HNF4α (1:100, goat, Santa Cruz Biotechnology SC-6556), and matching secondary anti-rabbit (1:500, donkey, A21207), anti-rat (1:500, chicken, A21472), anti-fluorescein isothiocyanate (1:1,000, rabbit, A11090) and anti-goat (1.500, chicken, A21468) with various fluorescent conjugates (all from Invitrogen). Confocal microscopy was performed on a Nikon A1 confocal laser microscope (Nikon Instruments, Melville, NY, USA) using a 20 × lens or 40 × and 60 × oil-immersion lenses. For some pictures and for quantification, four to six sections were merged. For macroscopic imaging, livers were visualized under a Leica MZ 16F fluorescent dissecting microscope. Immunoblotting Immunoblotting for Lrat, desmin or cytokeratin was performed on isolated primary hepatic cell populations using a mouse anti-Lrat antibody (dilution 1:5,000) [55] , desmin (Lab Vision, 1:2,000) and cytokeratin 19 (rat, Troma-III, 1:1,000, Developmental Studies Hybridoma Bank, University of Iowa). Briefly, cell or liver lysates were electrophoresed on 10% acrylamide SDS gels and transferred to nitrocellulose membrane. Loading was confirmed by Ponceau S staining. Blots were blocked in 5% non-fat dry milk, followed by overnight incubation at 4 °C with primary antibody, 1 h incubation with horseradish peroxidase-conjugated secondary antibody and detection by luminescence (SuperSignal, Thermoscientfic). Specificity of the Lrat antibody was determined using liver extracts from wild-type and Lrat knockout mice ( Supplementary Fig. S10C ). Blots were reprobed with actin antibody (1:5,000; MP Biomedicals) to confirm equal loading. Full-length images of all immunoblots are shown in Supplementary Fig. S10 . Quantification of positively stained cells HNF4α-positive hepatocytes were quantified in merged 20 × pictures representing 70–100 random 20 × fields per mouse. Three to four mice per treatment group were analysed. To determine Col-GFP-positive cells or αSMA-positive cells originating from HSCs, at least 50 random 40 × pictures were analysed per mouse. Experiments were performed in three to five animals per treatment group. Quantification of HNF4α-positive, αSMA-positive cells and Col-GFP-positive cells, and determination of co-localization with fluorescent Cre reporters were performed using ImageJ software. Statistical evaluation Statistical analysis was performed using Prism (GraphPad, San Diego, CA). Differences between two groups were calculated by Student’s t -test. Significance of differences between multiple groups was determined by one-way analysis of variance, followed by Dunnett’s post - hoc test. All data are expressed as means±s.d. How to cite this article: Mederacke, I. et al. Fate tracing reveals hepatic stellate cells as dominant contributors to liver fibrosis independent of its aetiology. Nat. Commun. 4:2823 doi: 10.1038/ncomms3823 (2013).